An RNA polymerase II-coupled function for histone H3K36 methylation in checkpoint activation and DSB repair Histone modifications are major determinants of DNA double-strand break (DSB) response and repair. Here we elucidate a DSB repair function for transcription-coupled Set2 methylation at H3 lysine 36 (H3K36me). Cells devoid of Set2/H3K36me are hypersensitive to DNA-damaging agents and site-specific DSBs, fail to properly activate the DNA-damage checkpoint, and show genetic interactions with DSB-sensing and repair machinery. Set2/H3K36me3 is enriched at DSBs, and loss of Set2 results in altered chromatin architecture and inappropriate resection during G1 near break sites. Surprisingly, Set2 and RNA polymerase II are programmed for destruction after DSBs in a temporal manner—resulting in H3K36me3 to H3K36me2 transition that may be linked to DSB repair. Finally, we show a requirement of Set2 in DSB repair in transcription units—thus underscoring the importance of transcription-dependent H3K36me in DSB repair. Eukaryotic genomes are constantly subjected to exogenous and endogenous forms of DNA damage [1] . Double strand breaks (DSBs) can lead to temporary loss of genetic information, and failure to repair DSBs can lead to severe genome instability and cell death. DSBs can be programmed (for example, meiosis and immunoglobulin rearrangements) or caused by exogenous agents (for example, ionizing radiation (IR), ultra-violet (UV) and anti-cancer drugs) [1] , [2] . In eukaryotes, chromatin plays a fundamental role in regulating the cellular response to DNA damage [2] . Among the factors that contribute to the DNA damage response (DDR) are histones and their post-translational modifications (for example, phosphorylated H2A serine 129; γ-H2A.X in metazoans), ATP-dependent chromatin remodellers (for example, RSC, INO80, TIP60), and histone variants (for example, Htz1) [2] . Transcription-associated histone modifications, including H3 lysine 4 methylation (H3K4me) and H3 lysine 79 methylation (H3K79me) also contribute to DDR and repair [2] . Interestingly, a majority of stalled replication sites tend to occur in transcribed genes [3] , increasing the propensity for the collision of transcription and replication bubbles eventually resulting in DSBs [4] . Yet, how the transcription apparatus influences DSB repair is not well understood. One major regulator of chromatin structure during transcription is H3 lysine 36 methylation (H3K36me). This mark is deposited by the Set2 methyltransferase and is highly conserved from yeast to humans [5] , [6] , [7] , [8] , [9] , [10] . Set2 is recruited, at least in part, through binding to hyper-phosphorylated RNA Polymerase II (RNAPII) after RNAPII enters the productive elongation phase [5] , [6] , [7] , [8] , [9] , [10] . Set2 recognizes the phosphorylated C-terminal domain (CTD) of RNAPII through the presence of a domain called the SRI domain (for S et2- R NAPII i nteraction domain) [7] , [8] . In yeast, Set2/H3K36me regulates chromatin structure in the bodies of genes by activating the histone deacetylase complex Rpd3S [5] , [11] , [12] , [13] and by regulating histone exchange through regulating the activity of Asf1, Chd1 and ISW1b complexes [14] , [15] . Outside of a role for Set2 in transcription elongation, much less is known regarding how this enzyme contributes to other DNA-templated functions. Here we describe a role for Set2/H3K36me in DNA repair, specifically repair of DSBs. We show that in budding yeast Set2/H3K36 is required for appropriate activation of the response to DSB as well as subsequent repair, a finding that is restricted to its function in transcription. Interestingly, we find that Set2 and RNAPII are programmed for destruction after DSBs, which for H3K36me, results in a temporal patterning of H3K36me2 and H3K36me3 around DSBs that we propose underlies the regulation of chromatin structure at break sites. Significantly, we find that Set2 loss leads to altered chromatin structure and inappropriate resection in G1 at break sites, which ultimately impacts pathway repair choice. Set2/H3K36me is required for resistance to DSB To test whether Set2 and H3K36me function in DNA damage repair, we assessed the sensitivity of yeast cells lacking SET2 to various genotoxic agents. Deletion of SET2 caused sensitivity to the DSB-causing agent phleomycin (an IR-mimic), mild sensitivity to the alkylating agent methyl methane sulphonate (MMS), but no sensitivity to hydroxyurea (replication stress) or UV (nucleotide damage) ( Fig. 1a ). The phleomycin sensitivity was rescued by transforming the set2Δ strain with full-length SET2 ( Fig. 1b ). In contrast, sensitivity of the set2Δ strain could not be suppressed by transformation with a catalytically inactive SET2 mutant ( SET2 H199L ); thus, methylation activity is required for survival after DSB ( Fig. 1b,f ). To further confirm the importance of Set2 in the DSB response, we utilized a strain (JKM179) in which a galactose-inducible, site-specific DSB in chromosome III can be repaired only by non-homologous end joining (NHEJ) [16] ( Fig. 1c ). Consistent with the phleomycin sensitivity found with deletion of SET2 , set2Δ was also sensitive to this galactose-induced DSB and was rescued by expressing wild-type (WT), but not catalytically inactive, Set2 ( Fig. 1c,d,f ). We ruled out the MAT -specific effect by using a strain with the homothallic ( HO ) endonuclease cut site in ADH4 gene and found that set2Δ was sensitive to a reparable Gal-inducible DSB as well ( Supplementary Fig. 1a ). Recently, it was suggested that Set2 functions in DNA damage in a catalysis-independent manner [17] ; however examination of the levels of H3K36me in the presumed C201A catalytic mutant used by Winsor et al. [17] revealed that it only abolished the tri-methyl form of H3K36 ( Supplementary Fig. 1b ). Importantly, and consistent with a role of Set2 methylation at H3K36 in this phenotype and DSB repair, we found that mutation of H3K36 (H3K36A) confers sensitivity to phleomycin ( Fig. 1e ). 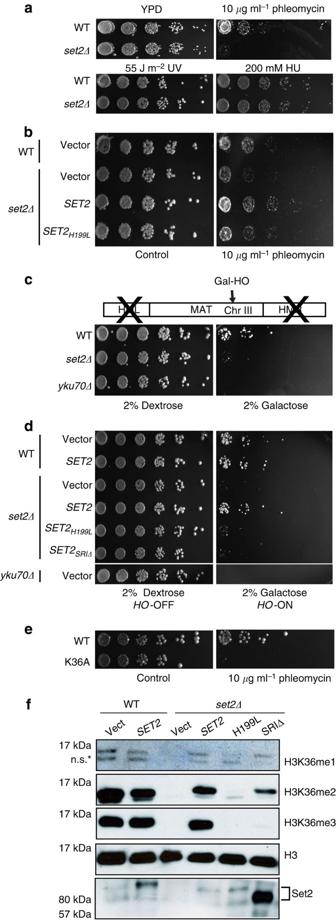Figure 1: Methylation by Set2 at H3K36 and RNAPII–Set2 interaction is required for cellular resistance against DSB. Fivefold serial dilutions of overnight cultures (grown either in YPD or appropriate selection medium for plasmids) were spotted on indicated plates and pictures were taken after 2–4 days. For immunoblots, log phase cultures were used for preparing whole-cell lysates as described in the ‘Methods’ section. (a) Aset2Δstrain is sensitive to phleomycin but not to hydroxyurea and UV. (b) Sensitivity ofset2Δto DSB can be rescued by WTSET2but not by a catalytically dead (SET2H199L) mutant. (c)set2Δis sensitive to persistent HO endonuclease-mediated DSB in the ‘donorless’ strain JKM179. Schematic of the ‘donorless’ strain is shown where the Gal-induced DSB is in theMATlocus of chromosome III. This strain has theHMLand theHMRdeleted and hence the DSB can be repaired only by NHEJ. (d) Rescue ofset2Δsensitivity to persistent DSB by WTSET2but not by a catalytically dead (SET2H199L) or the SRIΔ mutant. (e) H3K36A phenocopiesset2Δon phleomycin. (f) Immunoblots showing the expression from the constructs used inFig. 1b,d. All the experiments were replicated at least three times. Figure 1: Methylation by Set2 at H3K36 and RNAPII–Set2 interaction is required for cellular resistance against DSB. Fivefold serial dilutions of overnight cultures (grown either in YPD or appropriate selection medium for plasmids) were spotted on indicated plates and pictures were taken after 2–4 days. For immunoblots, log phase cultures were used for preparing whole-cell lysates as described in the ‘Methods’ section. ( a ) A set2Δ strain is sensitive to phleomycin but not to hydroxyurea and UV. ( b ) Sensitivity of set2Δ to DSB can be rescued by WT SET2 but not by a catalytically dead ( SET2 H199L ) mutant. ( c ) set2Δ is sensitive to persistent HO endonuclease-mediated DSB in the ‘donorless’ strain JKM179. Schematic of the ‘donorless’ strain is shown where the Gal-induced DSB is in the MAT locus of chromosome III. This strain has the HML and the HMR deleted and hence the DSB can be repaired only by NHEJ. ( d ) Rescue of set2Δ sensitivity to persistent DSB by WT SET2 but not by a catalytically dead ( SET2 H199L ) or the SRIΔ mutant. ( e ) H3K36A phenocopies set2Δ on phleomycin. ( f ) Immunoblots showing the expression from the constructs used in Fig. 1b,d . All the experiments were replicated at least three times. Full size image Set2 functions through its association with the elongating (phosphorylated) form of RNAPII [7] . We therefore investigated whether the DNA damage-induced phenotype we observed in the absence of Set2 and H3K36me is connected to its RNAPII function. We previously characterized a domain in the C terminus of Set2, termed the SRI domain, which is essential for coupling Set2 with the transcribing polymerase [7] . Mutation of this domain uncouples Set2 from RNAPII and results in selective loss of H3K36me3 ( Fig. 1f and ref. 18 ). Significantly, mutation of the SRI domain of SET2 (SRIΔ) could not rescue the sensitivity of set2Δ to persistent gal-induced DSB ( Fig. 1d ). Taken together, these data suggest that Set2 functions in DSB repair through its interaction with elongating RNAPII. They further suggest the possibility that transcribing polymerase itself may play an important role in DSB repair—a finding that would be consistent with studies showing RNAPII is present at DSBs [19] . SET2 is functionally connected to DSB response and repair To further establish that Set2 functions in cellular survival against genotoxic insults, we selected 30 genes representative of the pathways involved in DDR and repair and analysed double mutant sensitivity to MMS. We performed our genetic interaction screen using MMS because of its ability to activate several DNA repair pathways as compared with phleomycin, thus allowing us to initially capture more possible genetic interactions between SET2 and DDR genes. Our screen revealed that SET2 genetically interacts (both positively and negatively) with a subset of DDR and repair genes, albeit to different extents ( Fig. 2a and Supplementary Fig. 2a ). In addition to recapitulating some prior genetic interactions (for example, between SET2 and SLX5 ) reported by the Idekker group [20] , we discovered several novel genetic interactions upon MMS treatment (for example, RAD9 and RAD51 ) ( Fig. 2a ). We focused on DSB-specific genes and repeated the genetic interactions using phleomycin (examples shown in Fig. 2b and Supplementary Fig. 2a,b ). Interestingly, the set2Δrad9Δ double mutant was more sensitive to MMS and phleomycin than either single mutant alone, suggesting that Set2 functions in parallel to Rad9, to provide resistance to DSB ( Fig. 2a , and Supplementary Fig. 2c ). Like the set2Δ single mutants, the set2Δrad9Δ synthetic sickness was rescued by WT SET2 , but not by a catalytically dead version of SET2 ( SET2 H199L ) ( Supplementary Fig. 2c ). These results agree with similar findings recently reported in a high-throughput genetic interaction map using multiple genotoxic agents [21] . 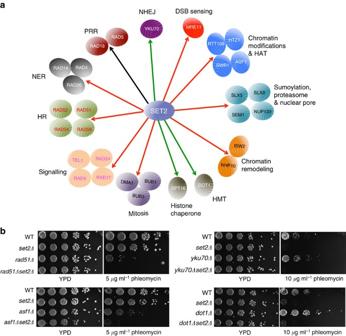Figure 2: Genetic interaction ofSET2with representative DDR and repair genes. Representative DDR and repair genes were selected from the Open Biosystems gene knockout collection and were verified by either phenotypic analysis or PCRs (using primers specific for the gene deletion) or both. Subsequent double mutants were made by gene replacement. (a) Qualitative representation of genetic interactions (on MMS) ofSET2with DDR and repair genes. Genes have been clustered together, manually, based on their annotated function in theSaccharomycesGenome Database (SGD). Black lines represent no genetic interaction, red lines indicate synthetic sick and green lines indicate same pathway interaction. The entire screen was repeated twice. (b) Serial dilutions of representative strains show thatset2Δis sick withrad51Δandasf1Δwhile theset2Δis epistatic to bothdot1Δandyku70Δon phleomycin. Individual spotting assays were done in triplicate plates (at once) and the set of triplicates were repeated twice. Figure 2: Genetic interaction of SET2 with representative DDR and repair genes. Representative DDR and repair genes were selected from the Open Biosystems gene knockout collection and were verified by either phenotypic analysis or PCRs (using primers specific for the gene deletion) or both. Subsequent double mutants were made by gene replacement. ( a ) Qualitative representation of genetic interactions (on MMS) of SET2 with DDR and repair genes. Genes have been clustered together, manually, based on their annotated function in the Saccharomyces Genome Database (SGD). Black lines represent no genetic interaction, red lines indicate synthetic sick and green lines indicate same pathway interaction. The entire screen was repeated twice. ( b ) Serial dilutions of representative strains show that set2Δ is sick with rad51Δ and asf1Δ while the set2Δ is epistatic to both dot1Δ and yku70Δ on phleomycin. Individual spotting assays were done in triplicate plates (at once) and the set of triplicates were repeated twice. Full size image As Set2 antagonizes the histone chaperone Asf1 to regulate histone exchange during transcription elongation [15] , we also investigated whether the sensitivity of set2Δ might be due to misregulated histone exchange after DSB. To test this, we analysed the asf1Δset2Δ double mutant on phleomycin. However, the double mutant was synthetically sick on phleomycin ( Fig. 2b ), indicating that Set2 is required for survival in the absence of Asf1 after DSB. Our data show that in regards to DSB, Asf1 and Set2 have independent functions. Since Set2/H3K36me is a histone modification associated with transcription elongation, we wondered whether any of the genetic interactions observed might be an indirect consequence of transcriptional alterations. However, transcription is only mildly affected in set2Δ (refs 22 , 23 ), and most of the changes are relatively modest increases in gene expression [23] . Notably, only a handful of genes are downregulated in set2Δ (shown in Supplementary Table 1 ), and do not include any canonical DDR or repair genes. Consistent with this, the gene expression and pathway analysis performed by Lenstra et al. [23] showed that set2Δ do not cluster with processes related to DDR and repair. Additionally, we investigated whether the protein levels of an early DSB response factor might be altered in set2Δ . We found no significant change in the proteins levels of yKu80, before or after DSB ( Supplementary Fig. 1c ). Thus, the specific sensitivity of set2Δ to DSB-causing agents is not attributable to an indirect effect of gene expression changes. Set2/H3K36me regulates checkpoint activation after DSB To determine whether the sensitivity of set2Δ was due to defective DNA-damage signalling, we exposed asynchronous cultures of WT and set2Δ strains to either MMS (M) or phleomycin (P) and monitored activation of γ-H2A.X (or H2AS129ph) and Rad53 (yeast homologue of mammalian Chk2). We observed reduced levels of Rad53 activation and γ-H2A.X in set2Δ , suggesting attenuated DSB damage response signalling ( Fig. 3a,b and Supplementary Fig. 3b ). Deletion of SET2 in the evolutionarily divergent yeast species Schizosaccharomyces pombe also resulted in reduced H2AS129ph when exposed to phleomycin ( Supplementary Fig. 3a ). 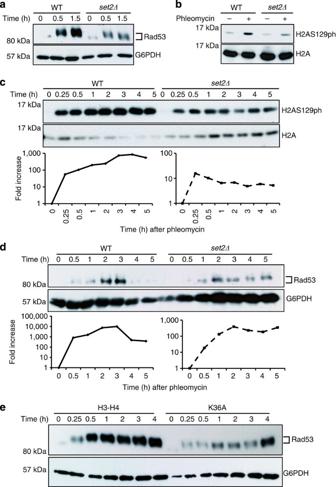Figure 3: DNA damage signaling is attenuated inset2Δ. Log-phase cells were exposed to phleomycin for indicated times and whole-cell extract was prepared (see Methods). (a) Diminution in Rad53 hyper-phosphorylation at indicated time-periods in aset2Δafter phleomycin treatment. The antibody to Rad53 is against the entire protein and G6PDH is used as a loading control. (b) Abrogated γ-H2A.X activation inset2Δafter phleomycin (50 μg ml−1) treatment for 2 hours. (c) Time-course showing the activation of γ-H2A.X after phleomycin treatment. Quantification (H2AS129ph/H2A) of the western blot is shown below. (d) Activation of Rad53 was monitored after phleomycin treatment in WT andset2Δ. Quantification (Rad53/G6PDH) of the western blot is shown below, which reveals abrogated DNA damage checkpoint activation inset2Δ(plotted as a semi-log plot). (e) H3K36A mutant cells also show abrogated DNA damage checkpoint activation as monitored by Rad53 activation kinetics. Representative western blots, from at least three biological replicates), are presented. Figure 3: DNA damage signaling is attenuated in set2Δ . Log-phase cells were exposed to phleomycin for indicated times and whole-cell extract was prepared (see Methods). ( a ) Diminution in Rad53 hyper-phosphorylation at indicated time-periods in a set2Δ after phleomycin treatment. The antibody to Rad53 is against the entire protein and G6PDH is used as a loading control. ( b ) Abrogated γ-H2A.X activation in set2Δ after phleomycin (50 μg ml −1 ) treatment for 2 hours. ( c ) Time-course showing the activation of γ-H2A.X after phleomycin treatment. Quantification (H2AS129ph/H2A) of the western blot is shown below. ( d ) Activation of Rad53 was monitored after phleomycin treatment in WT and set2Δ . Quantification (Rad53/G6PDH) of the western blot is shown below, which reveals abrogated DNA damage checkpoint activation in set2Δ (plotted as a semi-log plot). ( e ) H3K36A mutant cells also show abrogated DNA damage checkpoint activation as monitored by Rad53 activation kinetics. Representative western blots, from at least three biological replicates), are presented. Full size image γ-H2A.X activation is one of the earliest steps after DSB-induction and occurs with extremely fast kinetics [24] . To determine whether this reduced level of γ-H2A.X was due to inefficient activation or faster de-phosphorylation (which normally occurs later in the DDR pathway) [25] , we monitored the activation of γ-H2A.X after DSB induction by phleomycin. We observed significantly lower levels of γ-H2A.X within the first hour of phleomycin treatment of set2Δ cells ( Fig. 3c ), implying a function for Set2 at an early step after DSB. Additionally, and in line with reduced activation of DNA damage checkpoint, Rad53 hyper-phosphorylation was severely reduced in a set2Δ strain in a similar timescale ( Fig. 3d ). Importantly, we found Rad53 activation was also reduced in a H3K36A strain ( Fig. 3e ). Taken together, our data show that Set2-mediated H3K36me is essential for maximal activation of the DNA damage checkpoint after DSB induction. H3K36me2 and me3 are DSB-inducible and present at DSBs As the catalytic function of Set2 is responsible for providing resistance to DSBs ( Fig. 1 ) and full activation of DDR ( Fig. 3 ), we next determined whether the levels of H3K36me change after induction of DSB. We induced DSBs using phleomycin in an asynchronously growing culture and monitored H3K36me3 levels by western blot analysis. Interestingly, H3K36me3 levels increased globally within an hour after exposure to phleomycin and then returned to basal levels ( Fig. 4a ). In contrast, H3K36me2 increased with much slower kinetics ( Fig. 4b ) and reached its highest levels at a later time-point (that is, 4–5 h after phleomycin treatment). Although it is possible that the increase in H3K36me2 at the later time-point was an active response to DSB, the increase coincided with the decrease in H3K36me3—suggesting a specific loss of H3K36me3 to form more H3K36me2. To further verify that we were monitoring a DSB-inducible histone modification, we examined the levels of H3K36me3 near the site of DSB (0.2 kb distal to the DSB in the MAT locus) at early time-points to accurately capture a transient induction. H3K36me3 was increased, although modestly, within 30 min of galactose-induced DSB and tapered off ~75 min after DSB induction ( Fig. 4c ). This degree of increase is in line with the changes reported for H4 acetylation around the DSB [26] , [27] . Consistent with global H3K36me2 levels measured by immunoblot ( Fig. 4b ), ChIP analysis indicated that H3K36me2 was induced at a later time point than H3K36me3 ( Fig. 4d ). Further, we detected an enrichment of Set2 at the DSB at an early time-point following DNA damage ( Fig. 4e ). The specificities of our H3K36me3, H3K36me2 and Set2 antibodies were confirmed by inclusion of a set2Δ sample ( Fig. 4a–e and Supplementary Fig. 4 ). Collectively, our data indicates H3K36me3 is DSB-inducible and transitions into H3K36me2—a finding that coincides with transiently enriched Set2. 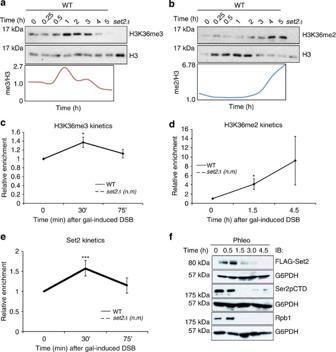Figure 4: Temporal regulation of H3K36me3 and H3K36me2 correlates with proteasome-mediated degradation of Set2. Immunoblots showing the levels of (a) H3K36me3 and (b) H3K36me2 after DSB induction by phleomycin. Exponentially growing yeast cells were exposed to phleomycin for indicated times and whole-cell extract was prepared. (c) H3K36me3 is transiently induced near the site of DSB (assessed by ChIP at 0.2 kb) at early time-points. The error bars represent ±s.e.m from two different biological replicates. n.m. represents ‘not measurable’ (d) H3K36me2 is induced near the site of DSB (assessed by ChIP at 0.2 kb), at later time points. The error bars represent ±s.e.m from two different biological replicates. * representsP<0.05 forcandd. (e) Preferential enrichment of Set2 near DSB (assessed by ChIP at 0.2 kb from DSB). *** representsP<0.01. (f) Time-course experiment after phleomycin treatment for Set2 (FLAG-Set2), Ser2pCTD (elongating RNA Polymerase II) and Rpb1 (largest subunit of RNAPII). G6PDH is used as loading control. Figure 4: Temporal regulation of H3K36me3 and H3K36me2 correlates with proteasome-mediated degradation of Set2. Immunoblots showing the levels of ( a ) H3K36me3 and ( b ) H3K36me2 after DSB induction by phleomycin. Exponentially growing yeast cells were exposed to phleomycin for indicated times and whole-cell extract was prepared. ( c ) H3K36me3 is transiently induced near the site of DSB (assessed by ChIP at 0.2 kb) at early time-points. The error bars represent ±s.e.m from two different biological replicates. n.m. represents ‘not measurable’ ( d ) H3K36me2 is induced near the site of DSB (assessed by ChIP at 0.2 kb), at later time points. The error bars represent ±s.e.m from two different biological replicates. * represents P <0.05 for c and d . ( e ) Preferential enrichment of Set2 near DSB (assessed by ChIP at 0.2 kb from DSB). *** represents P <0.01. ( f ) Time-course experiment after phleomycin treatment for Set2 (FLAG-Set2), Ser2pCTD (elongating RNA Polymerase II) and Rpb1 (largest subunit of RNAPII). G6PDH is used as loading control. Full size image To further understand the molecular basis for the temporal regulation of H3K36me2 and H3K36me3, we monitored the global levels of Set2 following DNA damage. Upon MMS and phleomycin treatment, we found that Set2 protein levels were significantly decreased ( Fig. 4f ). Surprisingly, we also noticed that the levels of Rpb1 (the largest subunit of RNAPII), and consequently the Ser2 phosphorylated form of RNAPII CTD (Ser2p CTD), also degraded after DNA damage in a proteasome-dependent manner ( Fig. 4f and Supplementary Fig. 4b,f ). Collectively, these results reveal a programmed destruction of Set2 and RNAPII after DSB, which may be an important event in DSB sensing and repair. To monitor whether we see a similar reduction in the levels of RNAPII in the vicinity of a DSB, we performed ChIP analysis for RNAPII around the MAT DSB. Consistent with the presence of Set2, we see RNAPII to be present at the same locus. Additionally, after 30 min of DSB induction, we can see significant reduction in the level of RNAPII ( Supplementary Fig. 4g ), a result consistent with our global analysis. To our knowledge, this is the first demonstration of proteasome-dependent regulation of RNAPII after DSB in any model system. To further understand how Set2 is regulated after DSB, we immunoprecipitated FLAG-tagged Set2 at several time-points following phleomycin treatment. We noticed an increase in pS/T-phosphorylation (a mark commonly associated with phosphorylation-dependent degradation [28] ) concomitant with reduced Set2 levels ( Supplementary Fig. 4d ). While Set2 degradation is likely attributed to loss of RNAPII interaction, an alternate hypothesis could be that Set2 is targeted for phosphorylation-dependent degradation in a checkpoint-dependent manner after DSB. However, we found that Set2 levels were still decreased in a number of key checkpoint mutants tested ( Supplementary Fig. 4e ). These data show that in WT cells, Set2, RNAPII and H3K36me are regulated after DSB, consistent with a role for Set2/H3K36me in regulating cellular resistance to DSB. Interplay between Set2 and chromatin regulators after DSB Our genetic and biochemical evidence suggests that Set2 has a methylation- and RNAPII-dependent function after DSB. Set2-catalysed H3K36me modulates chromatin structure via activation of the Rpd3S histone deacetylase complex [5] , [11] , [12] , [13] , antagonizing the function of Asf1 (ref. 15 ) and regulating ISW1b function [14] . Thus, we investigated whether any of these pathways contribute to the function of Set2 after DSB. As mentioned above, the asf1Δset2Δ double mutant is synthetically sick on phleomycin, suggesting that Set2 and Asf1 function in parallel after DSB ( Fig. 2b ). Consistent with this finding, we also noticed synthetic sickness of H3K36A with H3K56R (H3K56Ac being a marker of histone exchange) on phleomycin ( Supplementary Fig. 2e ). To test the other possible H3K36me effector proteins, we deleted RCO1 (Rpd3S-specific subunit), IOC4 (Isw1b-specific H3K36me effector protein) and YLR455w (a PWWP-containing putative H3K36me binder) and determined whether any of these strains phenocopied set2Δ . None of these known or putative H3K36me effector proteins showed similar phleomycin sensitivity as set2Δ in isolation ( Supplementary Fig. 2d ). Whether specific combinations of these effectors are required or whether a novel effector protein is reading H3K36me remains to be determined. We next investigated other histone modifiers known to play a role in the DDR, Dot1 and the histone variant Htz1. Dot1-dependent H3K79 methylation (H3K79me) and Htz1 are two chromatin components that are crucial for DSB response and repair [29] , [30] , [31] , [32] , [33] , [34] . H3K79me modulates the DSB checkpoint response by recruiting or stabilizing the Rad9 adaptor protein on chromatin [34] , [35] and inhibits DSB end-resection in a Rad9-dependent fashion [36] , [37] . Htz1 has been implicated in a multitude of events occurring after DSB. We investigated the genetic interactions between SET2 with DOT1 and HTZ1 to determine whether Set2 is part of any of the known pathways (or processes) in which these proteins function after DSB. We observed that set2Δ was synthetically sick with htz1Δ and swr1Δ ( Supplementary Fig. 2e ), but set2Δ suppressed the mild resistance of dot1Δ to phleomycin ( Fig. 2b ). These data reveal that Set2/H3K36me is required for cell survival in the absence of Swr1/Htz1 function. They also suggest that Set2 and Dot1 might function in antagonistic manner to regulate cellular response to DSB. Set2 regulates chromatin dynamics around a DSB Based upon synthetic sickness of set2Δ with genes involved in homologous recombination, early abrogation of DNA damage checkpoint and sensitivity to ‘error-prone NHEJ’ (as revealed by persistent DSB in JKM179 ‘donor-less’ strain) ( Fig. 1c ), we investigated whether the early steps of chromatin remodelling might be defective in cells deleted for SET2 . Thus, we induced DSB (in asynchronous cultures) by galactose treatment in the JKM179 donor-less strain and performed a time-course-based ChIP experiment for histones, their post-translational modifications and histone variants, at regions near the DSB and at an unrelated locus (ARS315) as a control. We monitored the DSB induction kinetics, using primers across the induced DSB, in WT and s et2Δ and found that to be identical ( Supplementary Fig. 5a ). We also confirmed the reduced DNA damage checkpoint activation in set2Δ by monitoring γ-H2A.X around a DSB. Consistent with previously published results for γ-H2A.X around a DSB, we observed a rapid accumulation of γ-H2A.X within an hour of DSB induction. In contrast, set2Δ showed no significant γ-H2A.X activation ( Fig. 5a ). 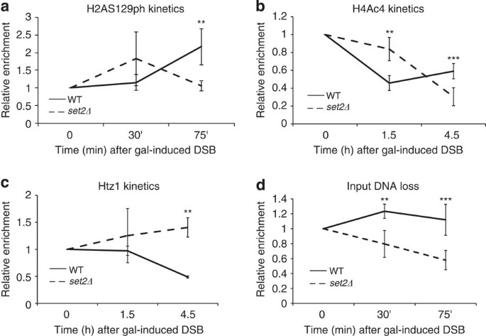Figure 5: Set2 regulates chromatin remodeling after DSB induction. (a) Reduced γ-H2A.X levels inset2Δby chip (** representsP<0.03; error bars show±s.e.m. from two independent biological replicates). (b) Altered kinetics of H4Ac4 at 0.2 kb from the DSB inset2Δat indicated time points (** representsP<0.03 and *** representsP<0.01; error bars show±s.e.m. from two independent biological replicates). (c) Increased Htz1 levels at 0.2 kb from the DSB inset2Δ(error bars represent mean±s.d. from two independent biological replicates). (d) Increased loss of input DNA inset2Δin G1-arrested cells at 1 kb away from the DSB (** representsP<0.03 and *** representsP<0.01; error bars show ±s.e.m. from two independent biological replicates). Figure 5: Set2 regulates chromatin remodeling after DSB induction. ( a ) Reduced γ-H2A.X levels in set2Δ by chip (** represents P <0.03; error bars show±s.e.m. from two independent biological replicates). ( b ) Altered kinetics of H4Ac4 at 0.2 kb from the DSB in set2Δ at indicated time points (** represents P <0.03 and *** represents P <0.01; error bars show±s.e.m. from two independent biological replicates). ( c ) Increased Htz1 levels at 0.2 kb from the DSB in set2Δ (error bars represent mean±s.d. from two independent biological replicates). ( d ) Increased loss of input DNA in set2Δ in G1-arrested cells at 1 kb away from the DSB (** represents P <0.03 and *** represents P <0.01; error bars show ±s.e.m. from two independent biological replicates). Full size image After a DSB, an early response of WT cells is to ensure a de-acetylated chromatin state, thereby enabling NHEJ in yKu70-80-dependent fashion [38] , [39] , [40] , [41] . Removal of yKu70-80, due to activation of Sae2 (and other resection enzymes) results in DSB being processed for homologous recombination [41] , which correlates with increased acetylation of histones [26] , [27] . Consistent with previously published results for H4 acetylation [38] , in WT cells, H4 acetylation decreased early, followed by an increase in H4 acetylation ( Fig. 5b , solid line, at 0.2 kb away from DSB). In contrast, H4 acetylation was significantly higher in set2Δ cells compared with WT cells around 1.5 h after gal-induced DSB ( Fig. 5b , dashed line). Notably, the subsequent increase in H4 acetylation seen in WT cells did not occur in set2Δ cells ( Fig. 5b , dashed line), indicating that the dynamic changes in H4 acetylation that normally occur after a DSB were altered in the absence of Set2—a result consistent with the idea that chromatin structure at DSBs is influenced by Set2 and H3K36me. As NuA4 drives, in large part, H4 acetylation at DSBs, the altered H4 acetylation seen in set2Δ cells may have been due to altered NuA4 activity (a result also consistent with the finding that NuA4 function is partially depended on H3K36me (ref. 42 )). Given the observed changes in H4 acetylation, we next looked at Htz1, an H2A histone variant that is deposited at DSBs by the SWR1 complex, which recognizes acetylated histones [43] , [44] , [45] . Consistent with published literature, Htz1 levels decreased in the vicinity of the DSB in WT cells ( Fig. 5c ; ref. 2 [2] ). In contrast, there was more retention of both Htz1 and H3 around the same DSB in set2Δ cells ( Fig. 5c and Supplementary Fig. 5b ). The level of Htz1 was not altered globally ( Supplementary Fig. 5f ). Aberrant retention of Htz1-containing nucleosomes around the DSB reduces the available biochemical pool of substrate for Tel1 (that is, H2A) and this may provide a molecular basis for the defects in the DNA damage checkpoint that is observed in the absence of Set2 (that is, reduced γ-H2A.X) ( Figs 3 and 6 ), although we formally do not rule out an abrogated activation of Tel1 as a molecular explanation. However, a similar antagonistic relationship has been observed in the case of ino80Δ (chromatin remodelling complex required for removing Htz1 from chromatin), where increased retention of Htz1 reduces γ-H2A.X (ref. 31 ). 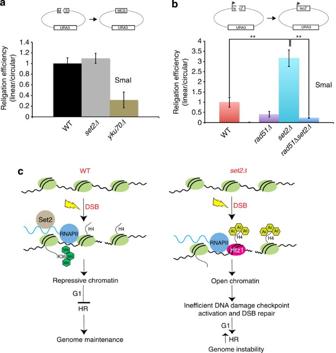Figure 6: Set2 primarily functions in DSB repair in the context of a transcribing unit. (a) Linearized (SmaI) or circularized pRS316 plasmids were transformed, in parallel, into the indicated strains and colony numbers were counted after 2–3 days on Sc-Ura plates. Religation frequency was calculated as the ratio of the number of colonies obtained from linearized plasmid to the number colonies obtained from circularized plasmid, with the value for WT strain normalized to 1.0.yku70Δis the positive control for the assay. (b) Linearized (SmaI) or circularized pGV255-live plasmids were transformed, in parallel, into indicated strains and number of colonies were counted after 2–3 days on Sc-Ura plates. Religation frequency was calculated as above (** representsP<0.02; error bars represent s.d. from three different independent transformation experiments). (c) A simplified model depicting a function of Set2 and H3K36me in regulating DDR and repair. Immediately after DSB (shown as ‘lightning bolt’), Set2-dependent H3K36me3 becomes enriched around the DSB. Increased H3K36me3 ensures a de-acetylated chromatin structure to prevent inappropriate DNA transactions especially in the context of a transcription unit, which we propose is important for maintaining the genomic integrity of transcribing units. Consistent with this model, loss of Set2/H3K36me leads to abrogated DNA damage signalling activation, altered chromatin structure and inappropriate repair. Figure 6: Set2 primarily functions in DSB repair in the context of a transcribing unit. ( a ) Linearized (SmaI) or circularized pRS316 plasmids were transformed, in parallel, into the indicated strains and colony numbers were counted after 2–3 days on Sc-Ura plates. Religation frequency was calculated as the ratio of the number of colonies obtained from linearized plasmid to the number colonies obtained from circularized plasmid, with the value for WT strain normalized to 1.0. yku70Δ is the positive control for the assay. ( b ) Linearized (SmaI) or circularized pGV255-live plasmids were transformed, in parallel, into indicated strains and number of colonies were counted after 2–3 days on Sc-Ura plates. Religation frequency was calculated as above (** represents P <0.02; error bars represent s.d. from three different independent transformation experiments). ( c ) A simplified model depicting a function of Set2 and H3K36me in regulating DDR and repair. Immediately after DSB (shown as ‘lightning bolt’), Set2-dependent H3K36me3 becomes enriched around the DSB. Increased H3K36me3 ensures a de-acetylated chromatin structure to prevent inappropriate DNA transactions especially in the context of a transcription unit, which we propose is important for maintaining the genomic integrity of transcribing units. Consistent with this model, loss of Set2/H3K36me leads to abrogated DNA damage signalling activation, altered chromatin structure and inappropriate repair. Full size image Given the critical role nucleosomal architecture plays in DSB response and the known role of FACT, a major regulator of nucleosome structure, in cellular resistance to DSBs in mammalian cells [46] , we next investigated whether SET2 functionally interacts with the FACT complex. Interestingly, the Spt16 subunit of FACT regulates H2A.X exchange at DSBs in human cells, indicating that FACT regulates nucleosome dynamics at DSBs. In yeast, mutants of Spt16 (for example, spt16-11 ) are sensitive to replication stress and high temperature and significantly, are suppressed by deletion of SET2 (refs 47 , 48 ). We therefore reasoned that FACT mutants may be sensitive to genotoxic agents and this genotoxic sensitivity would be suppressed by set2Δ . As shown in Supplementary Fig. 5c , we found that the spt16-11 allele was extremely sensitive to phleomycin at permissive temperature. Consistent with the idea that Set2 opposes the action of FACT function [48] , deletion of SET2 suppressed, albeit partially, the DSB sensitivity of the spt16-11 strain. These data suggest the intriguing possibility that Set2 and FACT have opposing effects on nucleosomal dynamics at DSBs. Set2 regulates DSB repair in the context of transcription We next investigated what the functional consequence of losing Set2 and H3K36me would be on DNA repair and repair pathway choice. Our data show that loss of Set2/H3K36me results in aberrant retention of Htz1-containing nucleosomes at DSBs, suggesting an unstable nucleosome architecture around these regions since Htz1-containing nucleosomes result in less stable nucleosomes [49] . Importantly, a recent study showed that Htz1-containing nucleosomes aid in Exo1-dependent end-resection [50] . We therefore used the input DNA from our cycling cells and monitored the loss of input DNA (as a surrogate readout of end resection). We did not detect any difference in the rate of input DNA loss compared with that of set2Δ cells ( Supplementary Fig. 5d ). However, end-resection is heavily influenced by the cell cycle (G1 versus G2/M), and smaller differences in resection kinetics may not become apparent in cycling cells. Therefore, we arrested cells in G1 by α-factor and monitored the loss of input DNA. In WT cells, we did not see any significant loss in input DNA, but, in set2Δ cells, the input DNA was rapidly lost, suggesting that set2Δ cells show faster end-processing in G1-arrested cells—a time when resection is normally suppressed ( Fig. 5d ). We confirmed this by monitoring the enrichment of single-strand DNA binding protein, RPA, in G1-arrested cells. We observed that even within 30 min after DSB induction, there is more RPA around a DSB in a set2Δ as compared with WT ( Supplementary Fig. 6a,b ). This effect is likely a direct consequence of having more Htz1-containing nucleosomes in a set2Δ as well as reduced γ-H2A.X, which is known to be inhibitory to resection [37] . One prediction from this observation would be that Set2 should regulate NHEJ, and in the absence of Set2, one should see lower end-joining efficiency. A canonical assay used to monitor the efficiency of end-joining is the calculation of the ratio of colony numbers obtained after transformation of linearized plasmids to that obtained from transforming a circular plasmid (that is, re-ligation efficiency). Using a plasmid where we generated a blunt-end cut in the plasmid multiple cloning site, we observed that there was no difference in the re-ligation efficiency between WT and set2Δ strains ( Fig. 6a ). However, since Set2 functions in the context of transcription units, we hypothesized that the function of Set2 in DNA repair would be more evident if our cut site was in the context of a gene body. We therefore carried out the plasmid re-ligation assay again, but in this case, with the cut site within the LacZ gene body. Strikingly, we observed a significant increase in plasmid re-ligation efficiency in set2Δ strains ( Fig. 6b ). We take these results to mean that although Set2 regulates pathway choice with a likely preference towards promoting NHEJ, the loss of Set2 does not completely ablate this function—hence, some plasmid would be re-ligated that would then serve as a template for ensuing HR as the balance has been tilted to this pathway. Importantly, HR is a canonical mechanism of repair in transcription units [51] , [52] , which would further exacerbate the set2Δ phenotype, resulting in more re-ligation. We next investigated whether this increased re-ligation efficiency is indeed a consequence of more recombination events, presumably due to transcription [51] . To answer that question, we deleted RAD51 in set2Δ and monitored the re-ligation efficiency. Consistent with the idea proposed above, we observed that the increase in plasmid re-ligation efficiency in a set2Δ was suppressed by deletion of RAD51 ( Fig. 6b ), indicating that set2Δ cells exhibit increased HR. To investigate whether this effect was specific for the type of DSB induced, we used another restriction enzyme (SacI) that creates staggered ends, again in the context of transcription. Even in this context, we observed higher plasmid re-ligation efficiency in set2Δ strains ( Supplementary Fig. 6c ). This phenotype of set2Δ is reminiscent of rsc and sth1 mutants, where linearization of the plasmid by digestion in a transcription unit resulted in higher re-ligation efficiency than WT cells [53] . Although the precise mechanism of increased re-ligation efficiency is not yet understood, these results reinforce the idea that Set2/H3K36me plays an important role in DSB repair, especially in the context of transcription. In this article, we provide genetic and biochemical evidence that Set2, and its methylation at H3K36, functions at an early step after DSB and plays a role in DSB repair. Specifically, we find Set2/H3K36me is critical for proper DSB checkpoint activation and impinges on pathway choice—results that can be linked to its function with elongating RNAPII. The role of Set2/H3K36me in DDR and repair is likely to maintain appropriate chromatin structure at break sites, which impinges on the molecular events that occur during DNA repair. Our data provide a temporal picture of how Set2 and H3K36me might modulate chromatin structure after a DSB. Using time-course immunoblotting and ChIP, we found that loss of Set2 leads to reduced γ-H2A.X, increased acetylation of H4 and aberrant retention of H3 and Htz1 at break sites. We propose that this altered chromatin architecture underlies the increased end-resection observed in G1-arrested cells, suggesting that HR is activated sooner in set2Δ at G1. Additionally, we found that loss of Set2 leads to increased HR, when a DSB is in the gene body. Future experiments will be required to determine whether H3K36me3 or H3K36me2 plays an important role in recruiting any DSB repair factors to control repair pathway choice, in a cell-cycle and/or transcription-dependent manner. Although H3K36me2 affects Ku70-80 recruitment to DSB in human cells [54] , such recruitment appears not to occur in cycling yeast cells as we did not see any significant alterations in Ku80 recruitment in set2Δ ( Supplementary Fig. 5e ). We found that Set2 and RNAPII are programmed for destruction after DSBs in a proteasome-dependent manner, which correlates with a transition of H3K36me3 to H3K36me2 ( Fig. 4 and Supplementary Fig. 4 ). Although the function of this transition in DSB repair is not yet known, we hypothesize that this methyl-state transition after DSB functions to ensure a chromatin structure that is temporally ‘tunable’ for DSB repair. We speculate that the fine-tuning of chromatin structure via H3K36me states would come from the ability of these different methyl states to activate/regulate functions of HATs and HDACs [55] . With regards to Htz1, the dynamic level of Htz1 around a DSB is critical for multiple steps in the response to DSB. Intriguingly, both in vivo and in vitro , H3K36me3 and Htz1 are mutually exclusive [56] , [57] ; hence, one function of an early increase in H3K36me3 at sites of DSBs could be to prevent Htz1 deposition, thereby allowing more H2A (H2A and Htz1 being mutually exclusive in chromatin) to be phosphorylated to form γ-H2A.X domains. Consistent with this idea, we observed increases in Htz1 and lower γ-H2A.X in a set2Δ ( Figs 3 and 5 ). Our study found that Set2’s function in DDR and repair is dependent on its association with elongating RNAPII ( Fig. 1 ). Consistent with this, we observed that when a DSB is in the context of transcription, deletion of SET2 leads to an increase in HR events ( Fig. 6 ). This result might be explained by the fact that Set2 loss tips the balance away from NHEJ to HR, which can be a preferred mechanism for break site repair in transcription units. We speculate that Set2-dependent chromatin compaction in G1 aids in preventing HR events, which would further prevent inappropriate recombination events that would arise in genes at this point in the cell cycle. It is also interesting to note that Set2/H3K36me is correlated with transcription rates and gene lengths [15] , which might fine-tune the appropriate type of repair that would occur in genes undergoing distinct rates of transcription. The dependence of Set2/H3K36me for proper repair in gene bodies provides further evidence for an RNAPII-dependent DNA damage-sensing mechanism. Lindsey-Boltz and Sancar [58] postulated the existence of such a DNA damage ‘sensor’ due to the extremely slow off-rate of RNAPII on DNA. Consistent with this idea, studies (including these herein) have found RNAPII at sites of DSB in yeast (and mammals) [19] and NuA4 and other chromatin modifiers that associate and function at DSBs are also associated with RNAPII [2] . In mammalian cells, DSB induces local chromatin silencing if the DSB is in a gene body. We surmise that the transcription machinery can be ‘co-opted’ by the DNA repair and signalling machinery to sense DNA damage and then use the already available chromatin modifiers (ATP-dependent remodellers/histone variants) to access and repair the damage, followed by restoration of the chromatin structure. This scenario would be especially useful during gene transcription induced R-loop formation, which can result in single or double-strand breaks [59] . Interestingly, both transcription and DSBs result in fairly identical mitotic recombination events [52] , making the possibility of RNAPII as a ‘constitutive DSB sensor’ even more plausible [58] . Given the stochastic nature of transcription [60] , using the transcription apparatus as a sensor for DNA damage can be a useful strategy for cells to rapidly respond to exogenous or endogenous genomic insults. Consistent with this model, a recent paper by the Legube group [61] shows that transcription units preferentially shunt the DSB to HR-dependent pathways. This phenomenon also was dependent upon the presence of the mammalian Set2 homologue, SETD2, and the presence of H3K36me3. We speculate that the DSB repair machinery can utilize the context-dependent chromatin environment to access and repair the DSB and maintain genome integrity. Finally, the conservation of H3K36me across different species lends credibility to the idea that H3K36me is also important for DSB repair and damage response in other organisms. Indeed, Tim Humphrey’s group [62] has discovered that the S. pombe Set2 also regulates pathway choice, because deletion of SET2 alters the balance between NHEJ and HR. Interestingly, they find that Gcn5 acetylates H3K36 (ref. 63 ) when Set2 is absent, and this activity leads to increased HR by presumably making the chromatin more accessible to the HR pathway. Additionally, Fnu et al. [54] showed that H3K36me2 catalysed by SETMAR/Metnase, which is not a canonical H3K36 methyltransferase, is critical for NHEJ in human cells. Taken together, we propose Set2 as a key player in the DNA repair pathway that likely impinges on genome stability. As human SETD2 [64] is mutated in a variety of cancers [65] , we speculate that SETD2 has a conserved role in DNA repair that would explain its connection to human disease. Yeast strains and plasmids All strains, unless otherwise stated, were in the BY4741 background. The strain for GAL -inducible HO endonuclease (JKM179) was obtained from James Haber, Brandeis University and subsequent gene deletions ( SET2 and YKU70 ) were performed by gene replacement using the PCR tool kit. The strains are listed in Supplementary Table 2 . Plasmids expressing SET2 from its own promoter were obtained from Scott Briggs (Purdue University) and the H199L mutation was made in full-length SET2 by site-directed mutagenesis (Quikchange, Stratagene). DNA damage sensitivity assays Cultures grown overnight were diluted to an OD 600 of 0.25, fivefold serially diluted and spotted on plates with or without relevant drugs. For UV experiments, cells were spotted on control plates and exposed to a range of UV dosage (from 20–60 J m −2 in Stratagene crosslinker P1800, rad4Δ served as a positive control for sensitivity to UV). For GAL -inducible DSB, overnight grown cells were serially diluted (starting ODs of between 2 and 5) as indicated above and spotted on Sc-Ura plates containing either 2% dextrose or 2% galactose. Pictures were taken after 2–4 days. For liquid culture experiments, log phase cultures were exposed to phleomycin (250 μg ml −1 except for Fig. 3b , wherein 50 μg ml −1 was used to test whether the phenotype was due to a high concentration of phleomycin) for indicated times, and then extracts were prepared by SUMEB method. About 5 O.D equivalent of cells were taken and lysed by bead beating using the lysis buffer containing (1% SDS, 8 M urea, 10 mM MOPS, pH 6.8, 10 mM EDTA, 0.01% bromophenol blue). In all, 200 μl of buffer with 200 μl equivalent of glass beads were used to lyse the cells. Bead beating was done for 6–8 min, intermittently, and the extracts were centrifuged, to clarify, and boiled at 95 °C for 5 min before loading the SDS–PAGE gel. Whole-cell protein extract and immunoblots Asynchronously grown mid-log (0.6–0.8 OD) phase cultures were lysed by SUMEB using glass beads, as mentioned above. For histones, 15% SDS–PAGE gels were run using Laemmli buffer. For Set2, RNA Polymerase II and Rad53 blots, 8% SDS–PAGE gels were run. Gels were transferred using a semi-dry Hoeffer apparatus at 45 mA per gel (constant current setting), 50 V for 1.5 h. For RNA Polymerase II, the Hoeffer setting was 55 mA per gel (constant current setting), 50 V for 1.5 h. Primary antibodies were incubated in 5% milk overnight and secondary antibodies were incubated in 5% milk for an hour. The immunoblots were developed using ECL-Prime from Amersham. An uncropped version of major immunoblots can be found in the Supplementary Fig. 7 . Antibodies: H3K36me1 (ab9048; 1:1,000); H3K36me2 (active motif 39255; 1:1,000 and 4 μl for ChIP), H3K36me3 (ab9050; 1:10,000 and 3 μl for ChIP), C-terminal H3 (EpiCypher 13-0001; 1:2,500 and 2 μl for ChIP), Set2 (raised in lab; 1:5,000 or 1:10,000 and 5 μl for ChIP), Rad53 (obtained from Daniel Durocher, Canada; 1:2,000 (for Fig. 3a ; ref. 66 ) and Abcam 104232; 1:2,000 (for all other Rad53 blots), H2AS129ph (Active Motif 39271; 1:1,000 and 2 μl for ChIP), H2A (Active Motif 39235; 1:25,000 and 2 μl for ChIP), G6PDH (Sigma; 1:100,000), Ser2pCTD (1:100, gift from Dirk Eick, LMU, Munich, Germany), Rpb1 (Santa Cruz, yN-18, 1:1,000), anti-Myc (9E10, 1:2,500), 4H8 against RNA Polymerase II (Active Motif; 1:10,000 and 4 μl for ChIP). Rabbit (Amersham, Donkey anti-Rabbit), goat and rat (both Jackson ImmunoResearch Laboratories) secondary antibodies was used at 1:10,000. RPA antibody (2 μl for ~1 mg of chromatin) from Valerie Borde (Insitut Pasteur, Paris, France) was used for ChIP in Supplementary Fig. 6 . ChIP JKM179 and derivatives thereof were grown overnight in YPD and the saturated culture was used to start a fresh culture in YEP lactate, pH 5.5 (SC-Ura plus 2% Sucrose for Fig. 5d ) at an OD 600 of 0.1 and grown at 30°C till the OD 600 reached 0.8–1.0. Galactose was added to a final concentration of 2% to induce the expression of HO endonuclease (at t =0 h). Samples were collected at required time-points and fixed with 1% (final concentration) formaldehyde. Cells were lysed using 300 mM FA lysis buffer (containing protease inhibitor cocktail). The lysed cells were sonicated (30% output, 6 pulses 6 times; 90% duty cycle) and clarified by centrifuging at full speed for 15 min. Immuno-precipitations were set up, overnight, with desired amount of proteins and antibodies (antibody amounts have been listed above). Protein G-sepharose beads (100 μl 1:10 diluted beads per 400 μl immunoprecipitation reaction) were added to the immuno-precipitation reactions and the reactions were allowed to incubate for 1 hour. Subsequent washes were done in 1.4 ml of 300 mM FA Lysis buffer, 500 mM FA-lysis buffer and LiCl solution (250 mM LiCl, 10 mM Tris, 0.5% each of NP-40 and sodium deoxycholate and 1 mM EDTA). The immunoprecipitates were resuspended in TE (pH 8.0) and treated with RNase for 30 min. The immunoprecipitates were then washed with TE (pH 8.0) and elution buffer was used to elute the DNA (15 min incubation in elution buffer followed by centrifugation at 3,000 r.p.m. for 2 minutes). The eluates were kept at 65°C overnight to carry out the de-crosslinking step and PCR purification kit (Qiagen) was used to extract the DNA. Details of PCR conditions, primer locations and analysis methodologies can be found in the Supplementary Methods . Immunoprecipitation Immunoprecipitation for Set2-FLAG was performed in accordance with the manufacturer’s protocol (SIGMA, catalogue no. A2220), using the 300 mM FA-lysis buffer used for ChIP experiments. MG-132 experiment Cells were grown in media containing proline as a nitrogen source overnight. The following morning, a fresh culture was started at OD 0.5 with 0.003% SDS and grown for 3 h before treatment with MG-132 (75 μM) for another 30 min. Subsequently, phleomycin (250 μg ml −1 ) was added and samples were obtained at indicated times, and western blotting was performed as described above. Plasmid re-ligation assay About 3–5 μg of circular plasmids were digested by indicated restriction enzymes. Running the digested plasmids on gels and performing routine gel extraction confirmed their linearization. Subsequently, 100 ng of linearized or circularized plasmids were transformed into indicated strains (LiAc/PEG method), in parallel. The colonies were counted on Sc-Ura plates after 2–3 days. Three independent transformation reactions were carried out. Statistical analysis For arriving at the P values in all the relevant experiments (ChIP assays and the plasmid re-ligation assay), we carried out unpaired Student’s t -test in Microsoft Excel. The explanations for the error bars are mentioned in the corresponding figure legends with relevant n values. P <0.05 was considered statistically significant. How to cite this article: Jha, D. K. et al. An RNA Polymerase II-coupled function for histone H3K36 methylation in checkpoint activation and DSB repair. Nat. Commun. 5:3965 doi: 10.1038/ncomms4965 (2014).